Commissural axonal corridors instruct neuronal migration in the mouse spinal cord Unravelling how neurons are guided during vertebrate embryonic development has wide implications for understanding the assembly of the nervous system. During embryogenesis, migration of neuronal cell bodies and axons occurs simultaneously, but to what degree they influence each other’s development remains obscure. We show here that within the mouse embryonic spinal cord, commissural axons bisect, delimit or preconfigure ventral interneuron cell body position. Furthermore, genetic disruption of commissural axons results in abnormal ventral interneuron cell body positioning. These data suggest that commissural axonal fascicles instruct cell body position by acting either as border landmarks (axon-restricted migration), which to our knowledge has not been previously addressed, or acting as cellular guides. This study in the developing spinal cord highlights an important function for the interaction of cell bodies and axons, and provides a conceptual proof of principle that is likely to have overarching implications for the development of neuronal architecture. Classical physiological studies have revealed a topographic map of neuronal activity, a major part of which is the stereotyped organization of neuronal cell bodies and the appropriate targeting of axons. Disruption of such organization is a well-known or inferred cause of neurodevelopmental disorders [1] . Thus, understanding how axons and neuronal cell bodies acquire the appropriate position has wide implications for both nervous system development and the underlying causes of neurodevelopmental disorders. During embryonic development, neurons migrate from the germinal zone, to acquire the correct adult spatial position, which is important for their connectivity [2] , [3] , [4] , [5] . Broadly, neuronal migration is thought to occur through two main modes; radial migration that involves neuronal cell bodies using radial glia as scaffolds (gliophilic migration) and tangential migration that is based on the response of cells to chemotactic cues [5] , [6] . As axons and neuronal cell bodies from different populations are guided simultaneously during development and are in close apposition, it seems plausible that forming axonal fascicles and cell bodies physically influence each other’s behaviour. A small number of studies have shown that the position of cell bodies influence the guidance of axons by the production of chemotactic cues [7] , [8] , [9] . Conversely, there is also evidence to support the idea that pioneer axons provide a growth substrate for newly migrating axons and cell bodies [10] , [11] , [12] . In addition, during a form of tangential migration, photographic evidence suggests that the migrating neuronal cell bodies appear as if they are using axons as migration scaffolds [5] , [6] , [13] , [14] , [15] . However, direct experimental evidence supporting the possibility of such neurophilic migration as a general mechanism remains sparse [5] , [16] , [17] , [18] , [19] , [20] . Moreover, experimental evidence supporting additional roles of axonal fascicles in neuronal migration other than neurophilic migration have not been defined. Despite the general significance of the interaction between axons and cell bodies during neuronal development, the vast majority of studies have investigated neuronal migration and axon guidance separately. How they influence each other’s behaviour thus remains poorly defined. In this study we address the issue of the developmental interaction between axonal fascicles and migration of cell bodies using the developing mouse ventral spinal cord as a model system. The developing ventral spinal cord is composed of motor neurons, which transmit motor information to the body and ventral interneurons that convey neuronal feedback to motor neurons and either directly or indirectly modulate motor activity [21] . Spinal commissural axons, many of which originate in the dorsal spinal cord, convey neuronal information between both sides of the body and project their axons through the ventral spinal cord before crossing to the other side of the nervous system ( Fig. 1 ) [22] . We find that ventral spinal interneuron populations migrate in a stereotyped pattern with respect to the forming commissural fascicles. This raises the possibility that commissural axons form fascicle ‘corridors’ that act as axonal neurophilic scaffolds and/or border landmarks to instruct neuronal migration. Here we show that profound disruption of commissural axonal routes by different molecular–genetic pathways ( Ntn-1 LacZ/LacZ and Dcc −/− and Robo3 −/− (refs 23 , 24 , 25 , 26 )) is correlated with aberrant cell body position. Whereas in a genetic mutant with mild commissural axonal defects, Boc −/− , no significant disruption is observed [23] . Moreover, we observe that reduction in the number of dorsally derived commissural neurons in chick embryos results in a concomitant change in the position of ventral interneuron cell bodies. Taken together, these data imply that the neuronal migration of ventral interneuron subsets are influenced by the presence of commissural axons at least in part in a cell non-autonomous way. To our knowledge, the finding that axons can act in a way other than as a permissive migration substrate has not been previously reported. These findings have broader implications for understanding how the development of axons and cell bodies from different populations of neurons interact to achieve a complex topographic network within the nervous system. 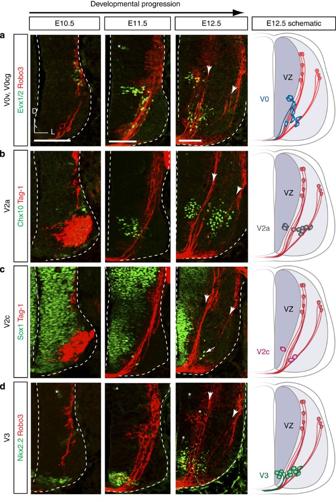Figure 1: Developmental time course of spinal ventral interneurons with respect to commissural axon projections. Transverse sections of E10.5–E12.5 mouse embryonic thoracic spinal cord immunolabelled with markers of commissural axons, Tag-1 and Robo3 (red), and markers of ventral interneuron populations (a) V0 (V0v and V0cg Evx1/2+), (b) V2a (Chx10+), (c) V2c (Sox1+) and (d) V3 (Nkx2.2+) (green). At least three embryos for each antibody/stage were analysed. Representative images are shown. Arrowheads point to the medial (left) and lateral (right) commissural fascicles at E12.5. Asterisk inaanddindicates artefactual antibody labelling. The small arrow incindicates the developing V2c, Sox1+ population in the mantle zone that distinguishes it from Sox1+precursors. White dashed lines indicate the outline of the spinal cord and lumen. Orientation label represents dorsal (D) and lateral (L). These data from E12.5 spinal cord are also represented as a schematic showing the medial and lateral commissural fascicle (red) and the relative spatial position of V0, V2a, V2c and V3. Scale bars, 100 μm (a) represent images from the same age/column of images. Figure 1: Developmental time course of spinal ventral interneurons with respect to commissural axon projections. Transverse sections of E10.5–E12.5 mouse embryonic thoracic spinal cord immunolabelled with markers of commissural axons, Tag-1 and Robo3 (red), and markers of ventral interneuron populations ( a ) V0 (V0v and V0cg Evx1/2 + ), ( b ) V2a (Chx10 + ), ( c ) V2c (Sox1 + ) and ( d ) V3 (Nkx2.2 + ) (green). At least three embryos for each antibody/stage were analysed. Representative images are shown. Arrowheads point to the medial (left) and lateral (right) commissural fascicles at E12.5. Asterisk in a and d indicates artefactual antibody labelling. The small arrow in c indicates the developing V2c, Sox1+ population in the mantle zone that distinguishes it from Sox1 + precursors. White dashed lines indicate the outline of the spinal cord and lumen. Orientation label represents dorsal (D) and lateral (L). These data from E12.5 spinal cord are also represented as a schematic showing the medial and lateral commissural fascicle (red) and the relative spatial position of V0, V2a, V2c and V3. Scale bars, 100 μm ( a ) represent images from the same age/column of images. Full size image Ventral neuron position is correlated with commissural axons To test the idea whether subsets of spinal ventral interneuron cell bodies could be influenced by commissural axons, we examined a developmental time course of ventral interneuron cell body migration with respect to the progression of commissural axonal fascicles in embryos ( Fig. 1 ). We first focused on mouse embryos where two robust markers are available to delineate commissural axons: Tag-1, which is a transient marker of early born motor and commissural axons, and Robo3, which, within the spinal cord, is a commissural axon-specific marker [22] , [24] . As described previously, two main commissural fascicles are apparent at mid-gestation ages: a medial fascicle that starts to form at mouse embryonic day E10.5 and expresses both Tag-1 and Robo3, and a lateral fascicle that expresses Robo3 more strongly than Tag-1 and is apparent later in development (from ∼ E12.5; Fig. 1 ) [22] , [27] . We examined the migration of cell bodies from both predominantly commissurally projecting neurons, V0 and V3 neurons, and V2a and V2c neurons, which are likely to be ipsilaterally projecting populations [28] , [29] , [30] , [31] , [32] , [33] . The nuclear position of these neuronal subpopulations were identified by transcription factor labelling, V0v/V0cg referred to in text as V0 (Evx1/2 + ), V2a (Chx10 + ), V2c (Sox1 + ) and V3 (Nkx2.2 + ) neurons [21] . We analysed a developmental progression of the migrating neuronal populations by examining progressively more developmentally advanced wild-type (WT) samples from E10.5 to E12.5 ( Fig. 1 ). Evx1/2 + V0 commissural neurons initially migrated laterally away from the ventricular zone and then turned and migrated ventrally along a path preconfigured by the pre-existing medial commissural fascicle ( Fig. 1a ) [29] . Chx10 + V2a neurons migrated in a medio-lateral direction coincident with radially oriented glial fibres ( Fig. 1b and Supplementary Fig. 1 ). At E12.5, V2a, neurons were segregated into two populations bisected by the medial commissural fascicle and delimited by the lateral commissural fascicle ( Fig. 1b ). To describe this phenomenon, we have coined the term ‘axon-restricted migration’. Sox1 + labels precursors in the ventricular zone and post-mitotic V2c neurons [28] . Sox1 + V2c migrated first through the medial commissural axon fascicle and then migrated ventrally on the lateral side of it to settle in a position close to the floor plate. Thus, once settled the V2c neurons were separated from the ventricular zone by the medial commissural axonal tract ( Fig. 1c ). Nkx2.2 + V3 neurons migrated initially in a medial–lateral direction, coincident with radial glial fibres, became separated into two groups bisected by the medial commissural fascicle and then occupied a dorso-lateral position within the ventral spinal cord ( Fig. 1d and Supplementary Fig. 1 ) [32] . Thus, for three of the four populations examined here, Chx10 + V2a, Sox1 + V2c and Nkx2.2 + V3 neurons, a pre-existing commissural fascicle appeared to form an apparent boundary defining the inner or outer limit for cell body populations in axon-restricted migration, whereas for Evx1/2 + V0 predominantly commissural neurons, the pre-existing medial commissural axonal tract preconfigured the ventral migration of Evx1/2 + V0 neurons. Commissural axon disruption leads to cell body misplacement The close stereotyped relationship between the forming commissural fibres and cell bodies of V0, V2a, V2c and V3 neurons lead us to consider that commissural axonal formation could influence cell body position. To examine this idea further, we analysed spinal cord interneuron cell body position in mouse embryos with known commissural axonal defects ( Fig. 2 ). The hypothesis that commissural axons influence cell body position would predict that abnormally positioned cell bodies would be observed following major disruption of commissural tracts, and that cell body positioning disruptions would be observed regardless of the causal molecular genetic manipulation as long as the commissural neurons were substantially disrupted. We therefore analysed mutant embryos caused by defects in different genes and with different degrees of commissural axon guidance phenotype severity ( Fig. 2 and Supplementary Fig. 2 ). We examined mouse mutant embryos with profound pre-crossing commissural axon guidance defects: Ntn-1 LacZ/LacZ (commonly known as Netrin-1 ), Dcc −/− ( Deleted in Colorectal Cancer , a known receptor of Netrin-1), Robo3 −/− and a genetic mutant with very mild commissural axonal defects, Boc −/− ( Figs 2 , 3 , 4 , 5 , 6 ) [23] , [24] , [25] , [26] . 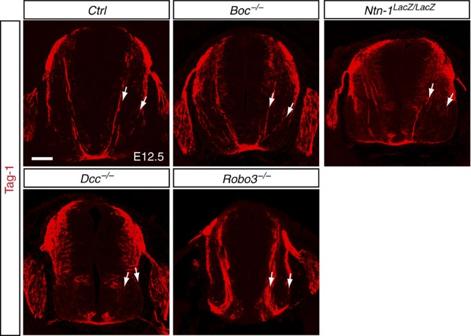Figure 2: Commissural axons are disrupted in unique ways inBoc,Ntn-1,DccandRobo3mutant embryos. Transverse sections of mouse E12.5 spinal cord in control,Boc−/−,Ntn-1LacZ/LacZ,Dcc−/−andRobo3−/−E12.5 embryonic sections immunolabelled with the commissural axon marker Tag-1 (red). The number of embryos examined forBoc−/−, Ntn-1LacZ/LacZ,Dcc−/−andRobo3−/−are 4, >6, >6 and 5, respectively. Representative images from this analysis are shown. The arrows point to the medial and lateral fascicles. Scale bar, 100 μm represents all images. Figure 2: Commissural axons are disrupted in unique ways in Boc , Ntn-1 , Dcc and Robo3 mutant embryos. Transverse sections of mouse E12.5 spinal cord in control, Boc −/− , Ntn-1 LacZ/LacZ , Dcc −/− and Robo3 −/− E12.5 embryonic sections immunolabelled with the commissural axon marker Tag-1 (red). The number of embryos examined for Boc −/− , Ntn-1 LacZ/LacZ , Dcc −/− and Robo3 −/− are 4, >6, >6 and 5, respectively. Representative images from this analysis are shown. The arrows point to the medial and lateral fascicles. Scale bar, 100 μm represents all images. 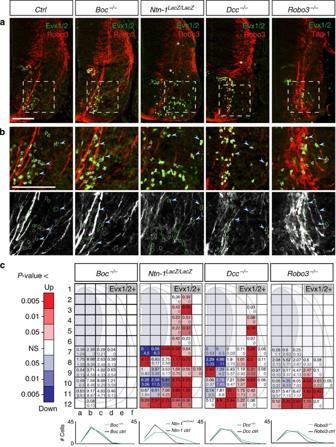Figure 3: V0 Evx1/2+interneuron cell body position is disrupted inNtn-1,DccandRobo3mutant embryos. (a,b) Transverse sections of control,Boc−/−(number of embryos quantified=4),Ntn-1LacZ/LacZ(n=6),Dcc−/−(n=6) andRobo3−/−(n=5) E12.5 embryonic spinal cord. (a) Representative images of E12.5 thoracic mouse spinal cord hemi-sections are shown. Immunohistochemical labelling with markers of commissural axons, Tag-1 or Robo3 (red), and the ventral interneuron population V0 (V0v and V0cg Evx1/2+: green) are shown as a merged images and as individual labelling. Asterisk inapoints to dorsally positioned V0 interneurons. The boxed areas inaare enlarged inb. Individual nuclei of neurons are outlined and arrowheads highlights interneurons associated with mis-projecting commissural axons. (c) Quantification of the phenotype. Images were captured and grids superimposed on the images (see Methods). The number of Evx1/2+neurons per bin were counted in two to six samples per embryo in mutant and control embryos (n=number of embryos quantified in mutant/control embryos) forBoc−/−(n=4/4),Ntn-1LacZ/LacZ(n=6/6),Dcc−/−(n=6/6) andRobo3−/−(n=5/5) embryos. Control groups were littermates of mutant embryos and therefore control groups were quantified separately forBoc−/−,Ntn-1LacZ/LacZ,Dcc−/−andRobo3−/−embryos. The average cell counts for mutant embryos (top left of each bin) and control embryos (bottom right) are indicated. The statistical variation relative to respective control embryos was determined using a one-tailed Student’st-test. Statistical significant differences between control and mutant embryos are presented as a heat map, with warm and cool colours representing a statistical increase or decrease from control values, respectively. These data are also presented with numericalP-values in theSupplementary Tables. Not significant changes are unchanged in colour from the background schematic. The medial–lateral average cell distribution for each population/genotype is depicted in graphical form underneath each schematic. Control (black line) and mutant (green line) embryo average cell counts are depicted. Thexaxis value is the summation of the average of all the bins within one column and theyaxis represents the total average cell number for each column. This graph therefore represents the overall medio-lateral distribution of each neuronal type/genotype. Scale bar, 100 μm (a,b) and represent all the images in that panel. Full size image Figure 3: V0 Evx1/2 + interneuron cell body position is disrupted in Ntn-1 , Dcc and Robo3 mutant embryos. ( a , b ) Transverse sections of control, Boc −/− (number of embryos quantified=4), Ntn-1 LacZ/LacZ ( n =6), Dcc −/− ( n =6) and Robo3 −/− ( n =5) E12.5 embryonic spinal cord. ( a ) Representative images of E12.5 thoracic mouse spinal cord hemi-sections are shown. Immunohistochemical labelling with markers of commissural axons, Tag-1 or Robo3 (red), and the ventral interneuron population V0 (V0v and V0cg Evx1/2 + : green) are shown as a merged images and as individual labelling. Asterisk in a points to dorsally positioned V0 interneurons. The boxed areas in a are enlarged in b . Individual nuclei of neurons are outlined and arrowheads highlights interneurons associated with mis-projecting commissural axons. ( c ) Quantification of the phenotype. Images were captured and grids superimposed on the images (see Methods). The number of Evx1/2 + neurons per bin were counted in two to six samples per embryo in mutant and control embryos ( n =number of embryos quantified in mutant/control embryos) for Boc −/− ( n =4/4), Ntn-1 LacZ/LacZ ( n =6/6), Dcc −/− ( n =6/6) and Robo3 −/− ( n =5/5) embryos. Control groups were littermates of mutant embryos and therefore control groups were quantified separately for Boc −/− , Ntn-1 LacZ/LacZ , Dcc −/− and Robo3 −/− embryos. The average cell counts for mutant embryos (top left of each bin) and control embryos (bottom right) are indicated. The statistical variation relative to respective control embryos was determined using a one-tailed Student’s t -test. Statistical significant differences between control and mutant embryos are presented as a heat map, with warm and cool colours representing a statistical increase or decrease from control values, respectively. These data are also presented with numerical P -values in the Supplementary Tables . Not significant changes are unchanged in colour from the background schematic. The medial–lateral average cell distribution for each population/genotype is depicted in graphical form underneath each schematic. Control (black line) and mutant (green line) embryo average cell counts are depicted. The x axis value is the summation of the average of all the bins within one column and the y axis represents the total average cell number for each column. This graph therefore represents the overall medio-lateral distribution of each neuronal type/genotype. Scale bar, 100 μm ( a , b ) and represent all the images in that panel. 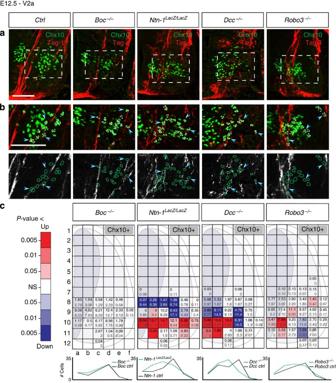Figure 4: V2a Chx10+interneuronal cell body position is disrupted inNtn-1,DccandRobo3mutant embryos. (a,b) Transverse sections of control,Boc−/−(number of embryos quantified=4),Ntn-1LacZ/LacZ(n=6),Dcc−/−(n=6) andRobo3−/−(n=5) E12.5 embryonic spinal cord. (a) Representative images from a ventral horn region from one side of a E12.5 thoracic mouse spinal cord are shown. Immunohistochemical labelling with markers of commissural axons, Tag-1 (red) and the ventral interneuron population V2a (Chx10+: green) are shown as merged images and as individual labelling. The boxed areas inaare enlarged inb. Individual nuclei of neurons are outlined and arrowheads highlight interneurons associated with mis-projecting commissural axons. (c) Quantification of the phenotype. The phenotype was quantified as described inFig. 3, Methods section and documented further in theSupplementary Tables 5–8. The schematic indicates where there is a statistically significant increase (red) or decrease (blue) in average cell number at that position. The graph shows the overall medial–lateral distribution of V2a neurons in control (black) and mutant (green) embryos. Scale bar, 100 μm (a,b). Full size image Figure 4: V2a Chx10 + interneuronal cell body position is disrupted in Ntn-1 , Dcc and Robo3 mutant embryos. ( a , b ) Transverse sections of control, Boc −/− (number of embryos quantified=4), Ntn-1 LacZ/LacZ ( n =6), Dcc −/− ( n =6) and Robo3 −/− ( n =5) E12.5 embryonic spinal cord. ( a ) Representative images from a ventral horn region from one side of a E12.5 thoracic mouse spinal cord are shown. Immunohistochemical labelling with markers of commissural axons, Tag-1 (red) and the ventral interneuron population V2a (Chx10 + : green) are shown as merged images and as individual labelling. The boxed areas in a are enlarged in b . Individual nuclei of neurons are outlined and arrowheads highlight interneurons associated with mis-projecting commissural axons. ( c ) Quantification of the phenotype. The phenotype was quantified as described in Fig. 3 , Methods section and documented further in the Supplementary Tables 5–8 . The schematic indicates where there is a statistically significant increase (red) or decrease (blue) in average cell number at that position. The graph shows the overall medial–lateral distribution of V2a neurons in control (black) and mutant (green) embryos. Scale bar, 100 μm ( a , b ). 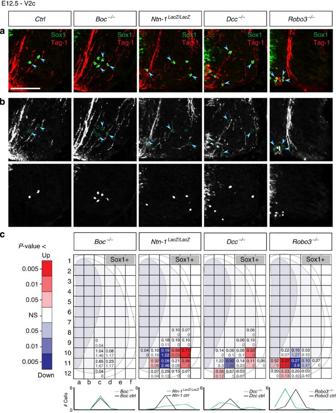Figure 5: V2c Sox1+interneuron cell body position is disrupted inNtn-1,DccandRobo3mutant embryos. (a,b) Transverse sections of control,Boc−/−(number of embryos quantified=4),Ntn-1LacZ/LacZ(n=6),Dcc−/−(n=6) andRobo3−/−(n=5) E12.5 embryonic spinal cord. Representative images from a ventral horn region from one side of a E12.5 thoracic mouse spinal cord are shown. Immunohistochemical labelling with markers of commissural axons, Tag-1 (red) and the ventral interneuron population V2c (Sox1+: green) are shown as merged image (a) and as individual labelling (b). Individual nuclei of neurons are outlined. Arrowheads highlights interneurons associated with mis-projecting commissural axons. Sox1 labelling to the left of the images are neuronal precursors in the ventricular zone. (c) Quantification of the phenotype. The phenotype was quantified as described inFig. 3, Methods section and documented further in theSupplementary Tables 9–12. The schematic indicates where there is a statistically significant increase (red) or decrease (blue) in average cell number at that position. The graph shows the overall medial–lateral distribution of V2c neurons in control (black) and mutant (green) embryos. Scale bar, 100 μm and applies to all images. Full size image Figure 5: V2c Sox1 + interneuron cell body position is disrupted in Ntn-1 , Dcc and Robo3 mutant embryos. ( a , b ) Transverse sections of control, Boc −/− (number of embryos quantified=4), Ntn-1 LacZ/LacZ ( n =6), Dcc −/− ( n =6) and Robo3 −/− ( n =5) E12.5 embryonic spinal cord. Representative images from a ventral horn region from one side of a E12.5 thoracic mouse spinal cord are shown. Immunohistochemical labelling with markers of commissural axons, Tag-1 (red) and the ventral interneuron population V2c (Sox1 + : green) are shown as merged image ( a ) and as individual labelling ( b ). Individual nuclei of neurons are outlined. Arrowheads highlights interneurons associated with mis-projecting commissural axons. Sox1 labelling to the left of the images are neuronal precursors in the ventricular zone. ( c ) Quantification of the phenotype. The phenotype was quantified as described in Fig. 3 , Methods section and documented further in the Supplementary Tables 9–12 . The schematic indicates where there is a statistically significant increase (red) or decrease (blue) in average cell number at that position. The graph shows the overall medial–lateral distribution of V2c neurons in control (black) and mutant (green) embryos. Scale bar, 100 μm and applies to all images. 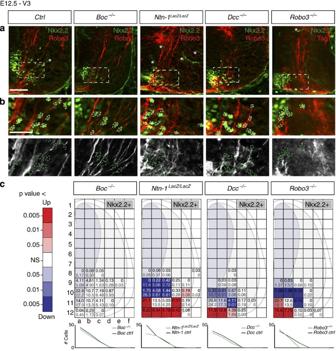Figure 6: V3 Nkx2.2+interneuron cell body position is disrupted inNtn-1,DccandRobo3mutant embryos. (a,b) Transverse sections of control,Boc−/−(number of embryos quantified=4),Ntn-1LacZ/LacZ(n=6),Dcc−/−(n=6) andRobo3−/−(n=5) E12.5 embryonic spinal cord. Representative images from a ventral horn region from one side of a E12.5 thoracic mouse spinal cord are shown. Immunohistochemical labelling with markers of commissural axons, Tag-1 or Robo3 (red) and V3 (Nkx2.2+: green) are shown as merged image and as individual labelling. Individual nuclei of neurons are outlined. The boxed area inais enlarged inbArrowheads highlight interneurons associated with mis-projecting commissural axons. (c) Quantification of the phenotype. The phenotype was quantified as described inFig. 3, Methods section and documented further in theSupplementary Tables 13–16. The schematic indicates a statistically significant increase (red) or decrease (blue) in average cell number at that position. The graph shows the overall medial–lateral distribution of V3 neurons in control (black) and mutant (green) embryos. Scale bar, is 100 and 50 μm (a,b), respectively. Full size image Figure 6: V3 Nkx2.2 + interneuron cell body position is disrupted in Ntn-1 , Dcc and Robo3 mutant embryos. ( a , b ) Transverse sections of control, Boc −/− (number of embryos quantified=4), Ntn-1 LacZ/LacZ ( n =6), Dcc −/− ( n =6) and Robo3 −/− ( n =5) E12.5 embryonic spinal cord. Representative images from a ventral horn region from one side of a E12.5 thoracic mouse spinal cord are shown. Immunohistochemical labelling with markers of commissural axons, Tag-1 or Robo3 (red) and V3 (Nkx2.2 + : green) are shown as merged image and as individual labelling. Individual nuclei of neurons are outlined. The boxed area in a is enlarged in b Arrowheads highlight interneurons associated with mis-projecting commissural axons. ( c ) Quantification of the phenotype. The phenotype was quantified as described in Fig. 3 , Methods section and documented further in the Supplementary Tables 13–16 . The schematic indicates a statistically significant increase (red) or decrease (blue) in average cell number at that position. The graph shows the overall medial–lateral distribution of V3 neurons in control (black) and mutant (green) embryos. Scale bar, is 100 and 50 μm ( a , b ), respectively. Full size image As reported previously, we observed important differences in the commissural axonal phenotype of Ntn-1 , Dcc , Robo3 and Boc mutant embryos, both in general commissural phenotype, as well as how one subset of transgenetically labelled medial commissural neurons, dI1 neurons, was selectively effected ( Fig. 2 and Supplementary Fig. 2 ) [23] , [24] , [25] , [26] , [34] , [35] . Boc mutant embryos were similar to WT with a relatively mild ( ∼ 5% previously reported widening) commissural defasciculation phenotype ( Fig. 2 ) [23] . In Ntn-1 mutant embryos, a clear medial commissural fascicle, including dI1 neurons, was observed, whereas other commissural fibres were highly defasciculated ( Fig. 2 ). In contrast, in Dcc mutant embryos the lateral commissural fascicle was apparently absent and the medial fascicle (including dI1 neurons) reduced and defasciculated ( Fig. 2 and Supplementary Fig. 2 ). The commissural neuron phenotype in Robo3 mutant embryos differs from that of Ntn-1 and Dcc mutant embryos, as in Robo3 mutant embryos commissural axons enter the ventral horn but in a defasciculated manner and unlike control embryos the medial Tag-1 + fascicle is not in close apposition to the ventricular zone ( Fig. 2 ). Although interplay between all pathways controlling commissural guidance is probable, this evidence supports the notion that each gene presented here plays a distinct role in the guidance of commissural neurons. We analysed neuronal cell body position in different mutant and control contexts by comparing averaged numbers of neurons in gridded bins (counting two to six samples from each of four to six embryos of each genotype; Figs 3 , 4 , 5 , 6 and Supplementary Tables 1–16 ). In E12.5 Boc mutant embryos, which, similar to WT, have a largely normal medial and lateral commissural fascicles, we did not observe any statistically significant differences in the position of V0, V2a, V2c and V3 neurons ( Figs 3 , 4 , 5 , 6 and Supplementary Tables 1, 5, 9 and 13 ). However, in mutants where the commissural neurons were severely disrupted ( Ntn-1 LacZ/LacZ , Dcc −/− and Robo3 −/− ), while the total number of neurons of each subtype examined was almost unanimously statistically indistinguishable regardless of genotype ( Supplementary Table 17 ), we observed profound and statistically significant change in neuronal position ( Figs 3 , 4 , 5 , 6 and Supplementary Tables 2–4, 6–8, 10–12 and 14–16 ). In Ntn-1 , Dcc and Robo3 mutant embryos, instead of migrating ventrally in a uniform stream, similar to mis-projecting commissural neurons, V0 neurons were mis-localized within the ventral horn that resulted in a statistically significant shift in neuronal position more laterally ( Fig. 3 and Supplementary Tables 2–4 ). Consistent with the notion that commissural axon tracts instruct the migration of V0 neurons, we observed a close association between the spatial positions of mis-located V0 cell bodies with those of misrouted Robo3 + commissural axons ( Fig. 3b ). In Ntn-1 LacZ/LacZ and, to a lesser extent, in Dcc −/− , and not in Robo3 −/− or control embryos, a statistically significant small number of V0 neurons were observed in a position dorsal to their dorsoventral birth height, suggesting they migrated dorsally instead of ventrally ( Fig. 3a and Supplementary Tables 2–4 ). By E12.5, control embryos formed two discrete nuclei of Chx10 + ipsilaterally projecting V2a neurons that appeared to be physically bisected by bundles of commissural axons ( Figs 1 and 4 ). Strikingly, in Ntn-1 , Dcc and Robo3 mutant embryos, V2a neurons generally formed a continuous mediolateral distribution with a statistically significant increased proportion of medially located Chx10 + cells ( Fig. 4 and Supplementary Tables 6–8 ). Thus, the mediolateral positioning of V2a neurons was profoundly disrupted in Ntn-1 , Dcc and Robo3 mutant embryos. However, radial glial fibres formed with a normal appearance in Ntn-1 , Dcc and Robo3 mutant embryos ( Supplementary Fig. 3 ). At 12.5, unlike control embryos, in Ntn-1 LacZ/LacZ and Dcc −/− embryos Sox1 + V2c neurons instead of clustering together in the ventral part of the ventral horn were spatially separated from each other and dispersed laterally within the ventral horn. Moreover, mis-localized Sox1 + V2c neurons appeared to be associated with laterally misplaced commissural fibres ( Fig. 5 and Supplementary Tables 10 and 11 ). In Robo3 mutant embryos, Sox1 + V2c neurons failed to migrate laterally but instead remained medial to the commissural fibres ( Fig. 5 and Supplementary Table 12 ). Nkx2.2 + V3 neurons, which, under control conditions, migrate out initially in a medio-lateral direction then pass the medial commissural fascicle, also failed to migrate out laterally in Robo3 , Dcc and Ntn-1 mutant embryos ( Fig. 6 and Supplementary Tables 14–16 ). Taken together, these data provide evidence that disruption of ventral interneurons cell body position is coincident with major disruption of commissural projections. Robo3 is not expressed in V2a Chx10 + or V2c Sox1 + neurons The finding that genetic disruption of Dcc , Ntn-1 or Robo3 results in ectopically placed cell bodies could be explained by at least two possible mechanisms; disruption of commissural neurons influenced the mis-migration of the ventral cell bodies (cell non-autonomous effect of commissural axons on ventral interneuron cell bodies) or that Dcc , Netrin-1 or Robo3 are expressed in the mis-migrating cell bodies themselves and the ectopic positioning of neurons is a direct result of loss of these genes within the responding cell body (cell autonomous effect). Dcc is broadly expressed and as there are many potential Netrin-1 receptors it is not possible to definitively exclude the possibility of the expression of such a receptor within these populations. Instead, we focused on Robo3 where there are clearly defined methods and tools for accurately determining its expression. Within the mid-gestation spinal cord, Robo3 has been reported to be selectively expressed in commissural neurons [24] . This suggests that in Robo3 mutant embryos, any effect on the cell body migration of ipsilaterally projecting populations, such as Chx10 + V2a and Sox1 + V2c neurons, would be as a result of disruption of commissural axons rather than the effected cell itself (a cell non-autonomous effect of commissural neurons on ventral cell bodies). To distinguish between these possibilities, first, by using in-situ hybridization and immunohistochemistry on consecutive sections we examined the expression of Robo3 messenger RNA in the Chx10 + and Sox1 + cell domains during the time they are undergoing their initial migration ( Fig. 7 ). We did not detect Robo3 transcripts in Chx10 + V2a or Sox1 + V2c neuronal regions at the stages examined ( Fig. 7 ). As this finding is a critical underlining element of our conclusions that the influence of commissural axons on neuronal migration is at least in part a cell non-autonomous effect, to verify this we also took an alternative approach. Green fluorescent protein (GFP) expression in Robo3 +/GFP heterozygote embryos labels cells that express or have a history of Robo3 gene activation. Thus, using confocal microscopy we examined whether there was coincidence of expression of GFP and Evx1/2, Chox10, Sox1 and Nkx2.2 in Robo3 +/GFP heterozygote embryos. Consistent with the above data, we observed GFP in Evx1/2 + V0 and medial Nkx2.2 + V3 neurons but not in Chox10 + V2a and Sox1 + V2c neurons in Robo3 +/GFP heterozygote embryos ( Supplementary Fig. 4 ). Taken together, these data support the notion that the mis-migration observed in Robo3 mutant embryos is at least in part a cell non-autonomous effect of disrupted commissural axons on cell bodies. 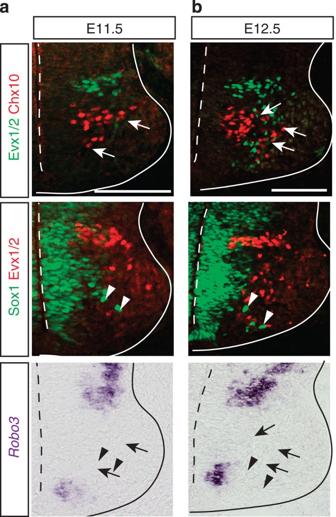Figure 7: Chx10+V2a and Sox1+V2c neurons do not expressRobo3at the time of initial migration. In-situhybridization and immunohistochemical labelling was performed on consecutive sections. Representative images showingRobo3mRNA (purple), V2a (red: Chx10+), V2c (green: Sox1+) and V0 (green or red: Evx1/2+) interneurons in transverse sections of WT (a) E11.5 (number of embryos (n)=3) and (b) E12.5 (n=3) embryonic spinal cord are shown. Arrows and arrowheads point to the position of Chx10+ V2a neurons and Sox1+V2c neurons, respectively. Continuous lines indicate the outline of the spinal cord; dotted line demarks the lumen of the spinal cord. Scale bars, 100 μm and represents images in the same column. Figure 7: Chx10 + V2a and Sox1 + V2c neurons do not express Robo3 at the time of initial migration. In-situ hybridization and immunohistochemical labelling was performed on consecutive sections. Representative images showing Robo3 mRNA (purple), V2a (red: Chx10 + ), V2c (green: Sox1 + ) and V0 (green or red: Evx1/2 + ) interneurons in transverse sections of WT ( a ) E11.5 (number of embryos ( n )=3) and ( b ) E12.5 ( n =3) embryonic spinal cord are shown. Arrows and arrowheads point to the position of Chx10+ V2a neurons and Sox1 + V2c neurons, respectively. Continuous lines indicate the outline of the spinal cord; dotted line demarks the lumen of the spinal cord. Scale bars, 100 μm and represents images in the same column. Full size image Dorsal spinal cord ablation leads to V3 neuron misplacement Taken together, this histological, genetic and expression evidence supports the notion that commissural axons influence the migration of ventral interneurons at least in part in a cell non-autonomous way. To test this idea further, we next adopted an alternative methodological approach using chicken embryos, which are particularly amenable to embryonic manipulation. The developing mouse and chick embryonic spinal cord are composed of largely equivalent neuronal subtypes, which develop in a comparable way [36] . In a number of higher vertebrates, including mouse and chick embryos, large cohorts of spinal commissural neurons are derived from the dorsal neural tube [37] . Therefore, a reduction of commissural neurons could be achieved by partial ablation of this region. We achieved this by expression of diphtheria toxin A (DTA) in one side of the dorsal spinal cord using electroporation and examined the effect on the position of neuronal cell bodies in the ventral spinal cord. The expression of DTA was regionally restricted by the 5′ addition of a HoxD4 enhancer to the expression plasmid that enriches expression in the dorsal neural tube ( Supplementary Fig. 5 ) [38] . We electroporated either control plasmids or a plasmid expressing DTA into chick embryos at around the onset of the first commissural axons, stage HH18, and analysed them at stage HH25 approximately equivalent to E11.5 in mouse embryos [37] , [39] . Analysis at later stages was not possible, as the only robust commissural axonal marker available in chick embryos, Axonin-1 (homologue of Tag-1 in mouse) becomes downregulated shortly after HH25 (ref. 39 ). Strict criteria were used for selection of samples for analysis that had simultaneous loss of the dorsal neural tube, while maintaining the cell number within ventral spinal cord ( Supplementary Fig. 5 ). Moreover, to avoid potential artefactual observations due to DTA being expressed in cells directly surrounding the neurons being examined or being affected by the distortion in the spinal cord caused by the ablation, we analysed the cell body position of V3 neurons, the most ventral neuronal population. Similar to mouse embryos, in chick embryos Nkx2.2 + V3 neurons are born in the most ventral part of the spinal cord, initially migrate out in a medio-lateral direction, through the medial commissural fascicle, and subsequently became segregated from the ventricular zone by the medial commissural fascicle before adopting a dorso-lateral position within the ventral spinal cord ( Supplementary Fig. 6 ) [32] , [40] . This suggests the general relationship between commissural axons and V3 neurons may be preserved between mouse and chicken embryos. Several consistent phenotypes were observed on the DTA -electroporated side compared with the unelectroporated (control) side of the same sample. As a consequence of ablation of cells in the dorsal spinal cord on the DTA-electroporated side of the embryo, a visible distortion in spinal cord shape was nearly always observed. Overall, a general reduction in the thickness of the Axonin-1 + medial commissural fascicle was observed on the DTA -electroporated side ( Supplementary Fig. 6 ). In the samples where this change in the thickness or positioning of the commissural fascicle was documented, we also observed an alteration in the positioning of Nkx2.2 + V3 neurons. In samples where on the control (unelectroporated) side a clear segregation of laterally located Nkx2.2 + V3 neurons to the ventricular zone was observed, on the DTA -electroporated side the size of this ‘gap’ was either observably reduced or no gap at all was apparent ( Supplementary Figs 5 and 6 ). In other cases, instead of being segregated by commissural axons, on the DTA -electroporated side the Nkx2.2 + V3 neurons were observed as intermingled with the remaining defasciculated commissural axons in a more dorsal position ( Supplementary Figs 5 and 6 ). To impose a quantifiable methodology for analysing these samples, we used the same counting method performed on mouse embryo samples above. However, in this electroporation experiment, a fundamental component of the experimental approach is partial ablation of the dorsal spinal cord resulting in distortion of the overall shape of the spinal cord, which could influence the outcome of this measurement. Nevertheless, using this method, we observed a statistically significant reduction in V3 neurons ventro-laterally positioned and an increase in dorso-medially located V3 neurons in the DTA-electroporated side compared with the non-electroporated side ( Supplementary Figs 5 and 6 ). This was not observed in embryos electroporated with control plasmids ( Supplementary Figs 5 and 6 and Supplementary Tables 18 and 19 ). Taken together, these data suggest that partial ablation of the dorsal neural tube results in reduction in commissural neurons and a concomitant change in the cell body position of ventrally located V3 neurons, which is consistent with the idea that commissural neurons instruct the migration of ventral interneuron cell bodies ( Fig. 8 ). 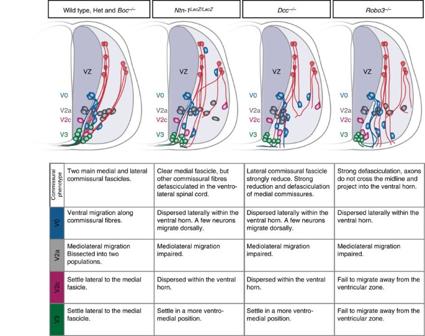Figure 8: Migration/axonal summary schematic. Schematic and tabular summary of the findings and conclusion showing the relationship between disruption of commissural axonal tracts (red) and ventral interneuron populations (V0, blue; V2a, grey; V2c, puce; and V3, green) in control,Boc,Ntn-1,DccandRobo3E12.5 embryonic spinal cord. Ventricular zone (dark purple/grey, VZ) and mantel zone (light purple/grey) are indicated. Figure 8: Migration/axonal summary schematic. Schematic and tabular summary of the findings and conclusion showing the relationship between disruption of commissural axonal tracts (red) and ventral interneuron populations (V0, blue; V2a, grey; V2c, puce; and V3, green) in control, Boc , Ntn-1 , Dcc and Robo3 E12.5 embryonic spinal cord. Ventricular zone (dark purple/grey, VZ) and mantel zone (light purple/grey) are indicated. Full size image We tested the idea that commissural fibre organization instructs the spatial arrangement of interneuronal cell bodies within the spinal cord. We found that individual subsets of spinal neurons have distinct migratory patterns with respect to commissural fibre formation. Furthermore, disruption of commissural axon position was coincident with neuronal migration defects that are at least in part due to a cell non-autonomous effect. Taken together, these data support the notion that commissural axons influence neuronal cell body positions ( Fig. 8 ). Our findings have general implications for the development of functional organization of the nervous system. A number of ligands such as Netrin-1 and their respective receptors have been shown to influence the migration of neuronal cell bodies by direct chemotactic mechanisms [41] , [42] . Our data supports an integrated mechanism of chemotropism and physical influences of axons on the positioning of neuronal cell bodies. We showed that a population of ventrally born Evx1/2 + V0 neurons ectopically migrated dorsally in Ntn-1 and Dcc but not in Robo3 mutant embryos suggests that loss of Netrin-1/Dcc-mediated ventral attraction in those neurons may have rendered them oversensitive to a ventrally located chemorepellant or dorsally located chemoattractant. However, our evidence suggests that in addition to classical chemotaxis, the physical arrangement of commissural axons also has a significant role in influencing cell body position, as the migration and positioning of neuronal cell body are highly stereotyped with respect to commissural axonal fascicles and severe disruption of commissural fascicle formation results in severe ventral spinal cord migration defects, independent of the genetic mutation that caused the commissural defect. This idea is supported further by the finding that the cell bodies of Robo3-negative ipsilaterally projecting neurons migrate aberrantly through loss of the commissural neuron-specific receptor Robo3 . There is good evidence to support the idea that in some contexts pioneer axons provide a growth substrate for newly migrating axons and cell bodies [10] , [11] , [12] . In addition, there are a number of reports of neuronal cell bodies that have the morphological appearance of migrating along axonal tracts [13] , [14] , [29] , [43] , [44] . For example, in the rat spinal cord, preganglionic cholinergic neurons have been shown to be in close apposition to commissural axonal tracts [14] , [43] , [44] . Despite the wide implications of neurophilic migration throughout the nervous system, little experimental work supports this model [16] , [17] , [18] . Moreover, apart from direct evidence of neurophilic migration in a small number of systems, other roles of axonal fascicles’ influence in neuronal migration have remained obscure. Taking advantage of the mouse mutants with known commissural guidance defects has enabled us to gain insight into how axonal fascicles instruct neuronal migration. Our evidence supports the idea that Evx1/2 + V0 neurons follow neurophilic migration, whereas V2a, V2c and V3 neurons appear to use commissural neurons as landmarks for segregation of these subpopulations in axon-restricted migration. Importantly, this is at least in part due to a cell non-autonomous effect of commissural axons on ipsilateral neuron cell bodies, as Robo3 is exclusively expressed in commissural neurons and V2a neurons are reported to be exclusively ipsilaterally projecting (not Robo3 expressing) neurons, yet are mis-localized in Robo3 −/− embryos [24] , [31] . Similarly, evidence points to V2c neurons being ipsilaterally projecting neurons, do not express Robo3 and are also are mis-localized in Robo3 −/− embryos [28] , [31] . Moreover, the finding that perturbation of dorsal commissural neurons by partial ablation of the dorsal spinal cord also results in mis-positioning of ventral interneuron cell bodies further supports this model. It is likely to be that all signalling pathways influencing commissural guidance integrate either directly or indirectly at some molecular level [45] . However, as we and others have demonstrated that Ntn-1 , Dcc , Robo3 and Boc mutant embryos have different neuronal phenotypes, this strongly supports partial non-overlapping functions of different genes in commissural guidance. We documented differences in the migration phenotypes between the different genetic mutant embryos examined in this study. DCC is a receptor of the ligand Netrin-1, yet the commissural axonal and migration phenotypes in Ntn-1 and Dcc mutant embryos are similar but not identical [25] . Several plausible explanations could account for this: first, several Netrin-1 receptors are known to be expressed in the developing spinal cord; therefore, Netrin-1 is modulating its effect via receptors in addition to DCC [46] , [47] , [48] , [49] . Second, Draxin, which is expressed in the developing spinal cord, was recently shown to be an alternative ligand for DCC [50] . Thus, DCC could be acting via a ligand in addition to Netrin-1. Third, Ntn-1 is a hypomorph and Dcc is a null mutation ( Supplementary Fig. 7 ). The commissural defects in the Robo3 mutant embryos are distinct from those observed in the Netrin-1/DCC pathway [24] . Unlike Ntn-1 and Dcc mutant embryos, V2c neurons of Robo3 mutant embryos failed to migrate out past the medial commissural fascicle. This could be accounted for by the observation that in Robo3 mutant embryos, in the most ventral part of the spinal cord, the commissural axons are misrouted further away from the newly differentiating V2c neurons than in the control embryos. In Robo3 mutant embryos, this may result in loss of contact between the commissural axons and newly formed V2c neurons, and therefore loss of an important instructive migratory cue. This suggests the possibility of direct cell–axon interactions influencing the migration of V2c neurons. Moreover, different subsets of commissural neurons are distinctly affected in Ntn-1 , Dcc and Robo3 mutant embryos. This, taken together with the finding that V0 neurons are differently affected in Ntn-1 , and Dcc and Robo3 mutant embryos, supports the general idea that an instructive cue on different subset(s) of commissural axons act as instructive guideposts for the migration of V0 neurons. Conversely, our evidence in the dorsal neuron ablation experiment, showing that reduction in the thickness of the medial commissural fascicle results in a smaller ‘gap’ between the V3 populations, implies that the size and position of this fascicle could be important to physically separate groups of V3 neurons. Overall, we favour the idea that both physical and instructive cues provided by commissural axons influence the positioning of ventral interneuron cell bodies. However, extensive experiments would be required to test this idea rigorously. Overall, our data suggests that the medial and lateral commissural fascicles have distinct roles in the position of cell bodies. Differential expression or presentation of adhesion molecules on commissural neurons and cell bodies could be responsible for the distinct influences on different types of commissural neurons. There is good evidence that adhesion molecules such as Tag-1 mediate neuronal migration, although it has, to date, not been possible to determine whether it is the adhesiveness of the cell body or axon that is the contributing factor [20] , [51] . Moreover, there are good examples of such differential adhesiveness regulating order in other parts of the nervous system, for example, retinal ganglion cell synaptic targeting within the brain, sorting of motor neurons pools within the spinal cord or dendritic self-avoidance [2] , [3] , [52] , [53] , [54] , [55] . Although such an ‘adhesion code’ has not been determined for commissural neurons, this is a plausible explanation to account for how different commissural axons could influence sorting of cell bodies. Taken together, our study provides evidence that axonal fascicles are an important machinery in the organization of spinal neuronal cell bodies. Our data support a role for commissural axons in neurophilic migration and, to the best of our knowledge, provide the first experimental evidence that commissural axonal fascicles act as border landmarks delimiting neuronal migration named ‘axon-restricted migration’. Several studies have shown that conversely, appropriate clustering of cell bodies can influence the axon to be guided appropriately [7] , [8] , [9] . Furthermore, it is well established that both axons and neuronal cell bodies are influenced by direct chemotactic mechanisms [5] . These previous studies integrated with the present study provide a concept of a tight interaction of cell bodies and axons that both physically influence each others guidance in a way that is integrated with classical chemotropism. Understanding how axons and cell bodies influence each other’s development has wide implications for understanding the assembly of functional organization within the nervous system. Animals and mouse embryos Netrin-1 LacZ/+ ( Ntn1Gt(pGT1.8TM)629Wcs ) (referred to as Ntn-1 LacZ/+ ) and Dcc +/− ( Dcctm1Wbg , RRID:MGI_MGI:3665466 ) mice were obtained from Professor Marc Tessier-Lavigne (Rockefeller University, NY, USA) and Professor Robert Weinberg (MIT, MA, USA), respectively [25] , [26] . A transgenic mouse line expressing GFP under the control of a Barhl2 enhancer Barhl2 GFP ( Tg(Barhl2-GFP)1Dodd ) was previously described [56] . The previously described Ntn-1 LacZ/+ line was generated by insertion of a gene trap vector containing β-galactosidase/neomycin cassette ( βgeo ) into intron 2, which together gives the possibility that a full-length WT Netrin-1 transcript with the βgeo cassette spliced out may be generated [26] . Using RT–PCR, we found that transcripts containing Netrin-1 coding exons 2–7 were size consistent with having spliced out the βgeo insert (3/3 embryos) in Ntn-1 LacZ/LacZ embryos ( Supplementary Fig. 7 ). Moreover, in-situ hybridization analysis using a probe to exons 3–7 revealed a low level of Netrin-1 exon 3 or beyond transcript in the Ntn-1 LacZ/LacZ embryos, albeit at a much reduced level ( Supplementary Fig. 7 ). This analysis supported the idea previously asserted that Ntn-1 LacZ/LacZ embryos were hypomorphs [26] . Genotyped Robo3 , Robo3;AtoZ + and Boc mutant mouse embryos were obtained from Professor Jane Dodd (Columbia University, New York, USA) and Professor Paola Bovolenta (CBM, Universidad Autonoma de Madrid, Spain), respectively. Mouse embryos were staged and processed as described previously [24] , [46] , [57] . Briefly, for genotyping genomic PCR, in-situ hybridization and/or epifluorescence (GFP) were used. The following previously described oligonucleotide primers were used in genotyping: GFP (GFP forward 5′-gca agc tga ccc tga agt tca-3′ and GFP reverse 5′-aac tcc agc agg acc atg tga-3′); β-galactosidase (LacZ-80 5′-gtc aat ccg ccg ttt gtt ccc acg g-3′ and LacZ-81 5′-gcg tgt acc aca gcg gat ggt tcg g-3′); DCC (DCC WT forward 5′-ggc cat tga ggt tcc ttt-3′, DCC WT reverse 5′-aag acg acc aca cgc gag-3′ and DCC mutant 5′-tcc tcg tgc ttt acg gta tc-3′); Neomyscin (Neo forward 5′-gga gag gct att cgg cta tga-3′ and Neo reverse 5′-ctt tct cgg cag gag caa ggt-3′). Ntn-1 Lcaz/LacZ embryos were genotyped by a vastly reduced level of Netrin-1 transcript detected by in-situ hybridization with the Netrin-1 exon 3–7 riboprobe (see below) [46] . Animal and experiments were performed according to institutional guidelines and national laws, and approved by the Ethical Committee for Animal Experiments for Northern Sweden. Both male and female adult mice of various ages were used to generate embryos of appropriate genotypes. Living mice were housed and kept under the routine high standards of care at Umeå University animal house. Of the embryos that were generated from our mouse colony, cervical dislocation was used to kill the female mice, to obtain embryos for experiments in this study. Reverse-transcriptase PCR RNA was extracted from mouse embryo tissue of Ntn-1 +/+ (number of embryo samples tested ( n )=4), Ntn-1 +/LacZ ( n =3) and Ntn-1 LacZ/LacZ ( n =4) embryos using the RNeasy miniprep kit (Qiagen), according to manufacturer’s instructions and complementary DNA synthesized using AccuScript High Fidelity 1st Strand cDNA Synthesis Kit (Agilent Technologies). RT–PCR was performed on samples, to amplify cDNA from Netrin-1 mRNA exons 2–7 (oligos: Netrin1exon2–7_for 5′-gtt gca agc cct tcc act ac-3′, Netrin1exon2–7_rev 5′- cag gcc caa aaa ttc aca gt-3′), and β-galactosidase (LacZ) (oligos: LacZ 80 and LacZ 81 described above). Plasmids and cloning The eukaryotic expression vector expressing a 5′ stop-lox GFP cassette was previously described [58] . The HoxD4-LacZ plasmid, which expresses β-galactosidase under the control of a HoxD4 enhancer element was previously described [38] . We cloned the region containing the HoxD4 enhancer, β-globin promoter, kozak sequence and start codon using XbaI/NcoI restriction enzyme sites into a plasmid containing CREpA in pBluescript, to produce a HoxD4-CRE plasmid. The HoxD4-DTA plasmid was generated by excising the HoxD4 enhancer (XhoI) from the HoxD4-LacZ plasmid and first cloning it into pBluescript ( HoxD4-bluescript ). The PGK-DTA-BGH poly-A fragment was excised from R26 mT/mG (Addgene plasmid 17787) using SalI and KpnI, and cloned downstream of the HoxD4 enhancer in HoxD4-bluescript using SalI and KpnI [59] . In-ovo electroporation White leghorn chicken eggs were obtained from Stellan Hennström, Vännäs, Sweden. Eggs were incubated at ∼ 38 °C for 3 days ( ∼ HH18), a time when the primitive spinal cord has formed but before significant commissural neuron differentiation has begun. The following DNA was injected into the lumen of the spinal cord. To examine the expression profile of the HoxD4 enhancer, the following plasmids were used: stop-lox GFP plasmid and HoxD4-CRE . To examine whether ablation of the dorsal spinal cord resulted in ventral neuron mis-migration, the following plasmids were used: control experiment (no ablation)— HoxD4-LacZ and pBluescript empty vector or HoxD4-LacZ and Barhl2GFP (a transgene to label dI1 neurons with GFP); experiment (ablation of the dorsal spinal cord)— HoxD4-LacZ and HoxD4-DTA or HoxD4-DTA and Barhl2GFP [56] . The spinal cord was then electroporated using a ECM830 electroporator (BTX, Harvard Apparatus) and BTX electrodes using 3 × 50 ms pulses at 30 V. Electroporated eggs were closed using electrical tape and subsequently incubated at ∼ 38 °C for a further 2 days and harvested at HH24–HH26, a time at which commissural axons are in close association with ventral interneurons and can be labelled with Axonin-1. Embryos were fixed in paraformaldehyde (4% w/v in PBS) on ice for 75 min, washed 3 × in PBS, equilibrated in sucrose solution (30% w/v in PBS) frozen in NEG-50 (Richard-Allan Scientific), gelatin or OCT compound (Sakura), sectioned and processed as described previously [57] . Immunohistochemistry Immunohistochemistry was performed as described previously [46] , [60] . Briefly, sectioned samples were blocked for 30 min at room temperature in blocking buffer (2.5% v/v heat-inactivated fetal bovine serum, in PBS—with or without 0.1% v/v Triton X-100). The primary antibody was incubated overnight at 4 °C in blocking buffer, washed 3 × for 5 min in PBS or PBS containing 0.1% v/v Triton X-100 and the secondary antibody incubated for 50 min to 3 h in blocking buffer at room temperature. The slides were then washed 3 × as described above, mounted and analysed. The following primary antibodies were used. The stock dilution for each antibody is indicated in brackets: rabbit: α-Axonin-1 (1:1,000) [39] , α-LH2 (1:1,000) [61] ,α-Sox1 (1:8,000) [57] , α-Chx10 (1:4,000) [62] , α-Tag-1 (1:10,000) [22] and α-Robo3 (1:1,000) [24] ; Guinea pig: α-Evx1/2 (1:8,000) [63] ; Mouse: Mab-Tag-1 (4D7) (1:6) [22] , Mab-Nkx2.2 (1:20), Mab-RC2 (1:50), Mab-HB9 (1:20) (Developmental Hybridoma) and Mab-Nestin (1:200) (Chemicon); and Chicken α-GFP (1:1,000) (Aves Labs) and α-β-galatosidase (1:1,000) (Aves Labs). Secondary antibodies were obtained from Jackson Immunochemicals. Fluorescein isothiocyanate, Cy3 and Cy5 secondary antibodies were used at the following concentrations 1:250, 1:1,000 and 1:500, respectively. In-situ hybridization In-situ hybridization was performed as described previously, using a digoxigenin-labelled riboprobe [64] . In short, samples were fixed in freshly prepared paraformaldehyde (4% w/v in PBS), washed in PBS (3 × 5 min), acetylated, washed in PBS (3 × 5 min) before prehybridizing at room temperature overnight in hybridization buffer (formamide (50% v/v) SSC (5 × ), bakers yeast RNA (250 μg μl −1 ), Denhart’s solution (5 × ) and herring sperm DNA (500 μg ml −1 )). cDNA plasmids were used to generate digoxigenin-labelled riboprobe to mNetrin-1 exons 3–7 and mRobo3 (refs 46 , 56 ). These probes were denatured (80 °C for 5 min and immediately cooled on wet ice) in hybridization buffer before being added to the sample. The slides were coverslipped and incubated in a humidified chamber at 70 °C for 24 h. The samples were sequentially washed in 5 × SSC (70 °C to remove the coverslip), 0.2 × SSC (70 °C for 1 h), B1 buffer (0.1 M Tris pH 7.5, 0.15 M NaCl ; to equilibrate at room temperature), incubated at room temperature in blocking buffer (blocking reagent (Roche); 2% w/v) in B1 buffer and incubated overnight at ∼ 4 °C with an alkaline phosphatase-conjugated antibody against digoxigenin (1:5,000 in blocking buffer; Roche). The samples were washed in B1 buffer (3 × 5 min) and then developed for 2 h to 3 days using 5-bromo-4-chloro-3-indolyl phosphate and 4-Nitro blue tetrazolium (Roche) at pH 9.5 at room temperature. Microscopy and image analysis Nikon Eclipse E800 fluorescence and LSM Zeiss 710 confocal microscopes were used. Brightness, contrast and gamma were adjusted in Adobe Photoshop CS4 and figures assembled in Adobe Illustrator. Quantification and statistical analysis of mouse embryos E12.5 embryonic spinal cord transverse sections were immunolabelled with Evx1/2, Chx10 and Sox1 in control, Boc −/− , Ntn-1 LacZ/LacZ , Dcc −/− and Robo3 −/− embryos. Control embryo were defined as WT, Boc +/− , Ntn-1 +/LacZ , Dcc +/− and Robo3 +/− heterozygote embryos. Sample size was chosen in line with the standard in the field. To minimize stage variation, Boc −/− , Ntn-1 LacZ/LacZ , Dcc −/− and Robo3 −/− embryos were compared with their own littermate controls, meaning that four separate control groups were quantified. The numbers of embryos quantified were as follows: Boc −/− (number of embryos quantified=4 mutants and 4 controls), Ntn-1 LacZ/LacZ ( n =6 mutants and 6 controls), Dcc −/− ( n =6 mutants and 6 controls) and Robo3 −/− ( n =5 mutants and 5 controls). Two to six samples for each embryo were quantified (see details in Supplementary Tables ). To quantify the neuronal distribution, images were captured from each embryo at an equivalent (thoracic) level. A 12 × 6 grid was superimposed on each image. To divide the area being analysed into normalized bins, the grid was stretched to conform to the dorsal and ventral, medial and lateral border of a half spinal cord (schematized in Figs 3 , 4 , 5 , 6 and Supplementary Tables ). The number of Evx1/2 + , Chx10 + , Sox1 + and Nkx2.2 + neurons in each bin were counted on each side of the spinal cord for each section. The mean distribution of neuronal number per bin was calculated for each mutant embryo and their respective controls (‘individual mean’). Values depicted in Figs 3 , 4 , 5 , 6 and Supplementary Tables 1–16 represent the average and s.d. of the ‘individual means’ of the same group (that is, neuronal population/genotype/bin position). Significant changes between ‘individual mean’ of control and mutant samples for each neuronal population/genotype/bin position were calculated using a one-tailed Student’s t -test assuming the variance are not equal. This test was specifically chosen, as the values cannot be assumed to follow a Gaussian distribution because ‘zero’ is a possible value included in the comparison. Without negative numbers, the distribution is more likely to move in one direction, thus the one-tailed test was used. The P -value associated with this relative increase or decrease in neuronal position in the mutant embryos is represented schematically by a colour code in Figs 3 , 4 , 5 , 6 (warm colours for an increase and cool colours for a decrease) and numerically described in Supplementary Tables 1–16 . As most samples were analysed in conjunction with commissural axonal labels, while all embryos were independently genotyped (see above), in some cases based on commissural axonal phenotype the investigators were aware of the genotype in advance of the cell counting analysis. Embryos analysed were of unknown and randomized sex. Selection and quantification of electroporated embryos We aimed to analyse samples in which DTA was expressed in the dorsal spinal cord, but importantly to avoid expression in the ventral spinal cord. This would permit analysis of the effect of cells derived from the dorsal spinal cord on ventral spinal cord neuronal migration. We used the HoxD4 enhancer to do this. First, to examine where the HoxD4 enhancer enriches expression after electroporation, we electroporated HH18 chick embryonic spinal cord with a lox-stop-lox-GFP plasmid and a HoxD4 CRE plasmid, and analysed them at HH25 ( Supplementary Fig. 5 ). GFP expression is therefore an indicator of where CRE under the control of the HoxD4 enhancer is expressed. The samples were sectioned in the transverse plane and imunolabelled with GFP (to indicate cells that have enhancer activity) and Nkx2.2 (to label V3 neurons), to see whether the GFP/enhancer activity overlapped with V3 neurons or was in close proximity. In the anterior thoracic spinal cord, the enhancer activity was generally restricted to the dorsal half of the spinal cord ( Supplementary Fig. 5a ). However, in some samples the expression spread further ventrally ( Supplementary Fig. 5a ). We considered these samples where the expression was detected more ventrally to be unsuitable. We concluded that although the HoxD4 enhancer was a useful tool to enrich expression in the dorsal spinal cord, this alone was not suitable for excluding expression in the ventral spinal cord. Therefore, for our data analysis, in addition to using the HoxD4 enhancer to enrich the expression of DTA to the dorsal spinal cord, we also set specific criteria for inclusion and exclusion of samples that required both a partial ablation of the dorsal spinal cord while maintaining the cell number in the ventral spinal cord. To do this, we imaged anterior thoracic sections from DTA- and control electroporated samples labelled with Hb9 (a general motor neuron marker at this age), Lh2 (a transcription factor that labels dorsally located dI1 neurons), Axonin-1 (which labels commissural axons) and Nkx2.2 (to label V3 neurons). These images were used to count the total number of Hb9 + , Lh2 + and Nkx2.2 + neurons on the electroporated (experiment) versus non-electroporated (control) side of the samples. For each image, the ratio of number of cells electroporated (experiment) versus non-electroporated (control) side was calculated for Hb9, Lh2 and Nkx2.2. This method assesses the total number of cells and not spatial position. For the DTA experiment, samples that were included in the analysis in this paper met the following criteria: first, the sections were from the anterior thoracic spinal cord level. Second, the ventral spinal cord including V3 neurons remained statistically similar in total cell number to the non-electroporated side. To assess this, the total number of the widely expressed motor neuronal marker HB9 and Nkx2.2, which labels V3 neurons, were counted and compared between control and electroporated sides. To be included in the analysis, the total number of HB9 + and Nkx2.2 + neurons on the electroporated side was at least 85% of the corresponding non-electroporated side. Third, a significant reduction in the dorsal spinal cord marker panLhx2/9 (Lh2) was observed on the electroporated side compared with the non-electroporated side (>50%; Supplementary Fig. 5 ). Samples that did not follow these strict criteria were discarded. To determine whether Nkx2.2 + V3 neuronal position was perturbed in this experiment, the number of Nkx2.2 + neurons were counted in gridded bins according to the method used for counting samples in the mouse embryos (see above). This statistical analysis was performed by comparing the cell number in the electroporated and non-electroporated side, using Student’s t -test ( Supplementary Figs 5 and 6 ). The sample size was similar to technically equivalent experiments in the field. The experiment was performed in three independent trials. This experiment statistical analysis contained seven DTA-electroporated embryos. Five of the seven DTA-electroporated embryos were analysed, as two of them did not meet the selection criteria for analysis. Six control embryos derived from two independent trials were used for quantification. Reduction of commissural neurons on the DTA-electroporated side was assessed by alteration in the pattern of the commissural axon label, Axonin1, and by the absence of expression of GFP (which labels dI1 commissural neurons in the experiments) on DTA-electroporated but not control electroporated embryos. As the DTA overexpression resulted in a large ablation that was morphologically visible in the samples, the investigators could distinguish the experimental and control sides in advance of the cell counting analysis. As with the mouse experiment, a standardized binning and counting method was imposed. However, unlike the mouse experiment, the overall distortion of the spinal cord could influence the outcome of this experiment. As with the mouse experiment, the embryos analysed were of unknown and randomized sex. How to cite this article: Laumonnerie, C. et al . Commissural axonal corridors instruct neuronal migration in the mouse spinal cord. Nat. Commun . 6:7028 doi: 10.1038/ncomms8028 (2015).